Observation of strong electron pairing on bands without Fermi surfaces in LiFe1−xCoxAs In conventional BCS superconductors, the quantum condensation of superconducting electron pairs is understood as a Fermi surface instability, in which the low-energy electrons are paired by attractive interactions. Whether this explanation is still valid in high- T c superconductors such as cuprates and iron-based superconductors remains an open question. In particular, a fundamentally different picture of the electron pairs, which are believed to be formed locally by repulsive interactions, may prevail. Here we report a high-resolution angle-resolved photoemission spectroscopy study on LiFe 1− x Co x As. We reveal a large and robust superconducting gap on a band sinking below the Fermi level on Co substitution. The observed Fermi-surface-free superconducting order is also the largest over the momentum space, which rules out a proximity effect origin and indicates that the order parameter is not tied to the Fermi surface as a result of a surface instability. Two main categories of theoretical descriptions arise when trying to describe the high- T c superconductivity of the iron-based superconductors (IBSCs): the weak coupling approach, which involves only the low-energy electronic structure near the Fermi level ( E F ) (refs 1 , 2 , 3 , 4 , 5 ), and the strong coupling approach, which emphasizes the local magnetic moments and strong Coulomb interactions [6] , [7] , [8] , [9] , [10] . In the former, superconductivity emerges as a Fermi surface (FS) instability and is, in principle, sensitive to FS changes. In particular, the superconducting (SC) gap is tied to the FS and its amplitude is strongly influenced by the nesting conditions. In the latter, the pairing is caused by local antiferromagnetic exchange couplings, well defined in the real space, which lead to a SC order parameter (OP) that is fixed in the momentum space and relatively insensitive to small changes of the electronic structure near the FS. In principle, one can distinguish between these two approaches and get critical information on the pairing mechanism of IBSCs by tracking precisely the evolution of the SC OP on bands for which the contributions to the FS vary drastically. In this respect, LiFe 1− x Co x As offers a perfect platform for this study because it undergoes a Lifshitz transition with one FS disappearing at small Co substitution [11] , [12] . Here we show a high-resolution angle-resolved photoemission spectroscopy (ARPES) study on SC LiFe 1− x Co x As. We reveal a large and robust SC gap with 2Δ α / k B T c ~7 on the inner hole band that is sinking below the Fermi level on Co substitution. The observed FS-free SC gap is also the largest over the momentum space, which rules out a proximity effect origin and indicates that the SC OP is not tied to the FS as a result of a FS instability. FS topology of pristine LiFeAs and LiFe 0.97 Co 0.03 As We first look at the FS topologies of pristine LiFeAs and LiFe 0.97 Co 0.03 As, which are illustrated in Fig. 1 . In agreement with previous studies, the substitution of Co introduces electron carriers and effectively moves the chemical potential upwards [11] , [12] , [13] , [14] . Since the inner hole-like FS (the α FS) shown in Fig. 1a only barely crosses E F in pristine LiFeAs [15] , [16] , a slight substitution of Fe by Co removes this tiny FS pocket at the Γ(0,0) point, and thus the system undergoes a Lifshitz transition [12] . The remnant intensity at E F around Γ in Fig. 1b is attributed to the limited energy resolution setting (~14 meV) for this normal state (NS) measurement ( T =30 K), which broadens the spectral width beyond E F . 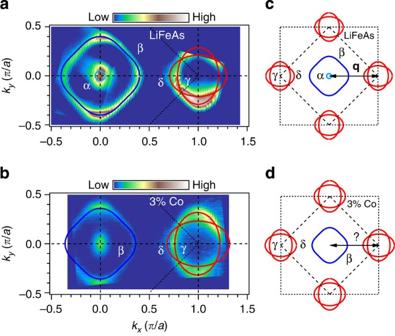Figure 1: FS topology of pristine LiFeAs and LiFe0.97Co0.03As. (a,b) Plots of the ARPES intensity atEFof LiFeAs (Tc=18 K) and LiFe0.97Co0.03As (Tc=15 K) as a function of the two-dimensional wavevector measured at 30 K with the He Iα (hν=21.218 eV). The intensity is obtained by integrating the spectra within 10 meV with respect toEF. (c,d) ExtractedkFloci of LiFeAs and LiFe0.97Co0.03As, respectively. The small hole-like FS at the BZ centre is sinking belowEFdue to the Co substitution and expected to significantly suppress the interband scattering between the electron and hole FSs. Figure 1: FS topology of pristine LiFeAs and LiFe 0.97 Co 0.03 As. ( a , b ) Plots of the ARPES intensity at E F of LiFeAs ( T c =18 K) and LiFe 0.97 Co 0.03 As ( T c =15 K) as a function of the two-dimensional wavevector measured at 30 K with the He Iα ( hν =21.218 eV). The intensity is obtained by integrating the spectra within 10 meV with respect to E F . ( c , d ) Extracted k F loci of LiFeAs and LiFe 0.97 Co 0.03 As, respectively. The small hole-like FS at the BZ centre is sinking below E F due to the Co substitution and expected to significantly suppress the interband scattering between the electron and hole FSs. Full size image Band dispersions of LiFe 1− x Co x As near E F To accurately determine the band top of the α band, we performed high-resolution (~3 meV) ARPES measurements in the vicinity of Γ for samples at three doping levels ( x =0, 1%, 3%, with onset T c ≈18, 16, 15 K, correspondingly, as shown in Supplementary Figs 1 and 2 ). As seen in Fig. 2d–f , the band top shifts to 4 and 8 meV below E F at Co contents of 1 and 3%, respectively. This shift is also clearly demonstrated by the energy distribution curves (EDCs) shown in Fig. 2m–o . While the low-energy quasiparticle peaks of pristine LiFeAs are clearly cutoff by the Fermi-Dirac (FD) function, those of the 1% Co and 3% Co samples shift below E F with small spectral weight at E F due the finite peak width. 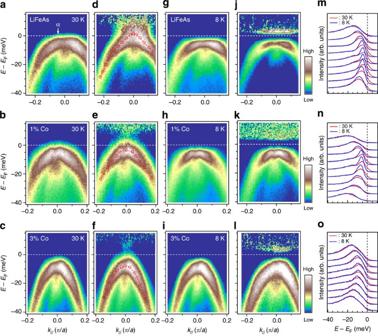Figure 2: Band dispersions of LiFe1−xCoxAs nearEF. (a–c) ARPES intensity plots of pristine LiFeAs, 1% Co and 3% Co samples, respectively, in the NS across the BZ centre. The data are recorded with the He Iα line (hν=21.218 eV), which is close tokz=0. (d–f) Same data as ina–c, but divided by the FD function convoluted with the system resolution. Red circles are the extracted NS dispersion of the α band. The α band is sinking belowEFin the 1% Co and 3% Co compounds. (g–i) Corresponding intensity plots in the SC state. (j–l) Same data as ing–i, but divided by the FD function convoluted with the system resolution. The difference between the NS and the SC state is clearly resolved (m–o), where the representative EDCs in both the NS and the SC state are plotted together. The enhanced spectral weight at the low binding energy is attributed to the coherence of the paired electrons. Figure 2: Band dispersions of LiFe 1− x Co x As near E F . ( a – c ) ARPES intensity plots of pristine LiFeAs, 1% Co and 3% Co samples, respectively, in the NS across the BZ centre. The data are recorded with the He Iα line ( h ν =21.218 eV), which is close to k z =0. ( d – f ) Same data as in a – c , but divided by the FD function convoluted with the system resolution. Red circles are the extracted NS dispersion of the α band. The α band is sinking below E F in the 1% Co and 3% Co compounds. ( g – i ) Corresponding intensity plots in the SC state. ( j – l ) Same data as in g – i , but divided by the FD function convoluted with the system resolution. The difference between the NS and the SC state is clearly resolved ( m – o ), where the representative EDCs in both the NS and the SC state are plotted together. The enhanced spectral weight at the low binding energy is attributed to the coherence of the paired electrons. Full size image Although the electronic structure of LiFe 1− x Co x As is quite two dimensional, previous studies indicate that the α band has a small dispersion along k z (refs 11 , 12 , 16 ). To quantify the k z effect of the α band and confirm that it does not cross E F along k z , we extract the NS dispersion of the α band at k z =0 and π . 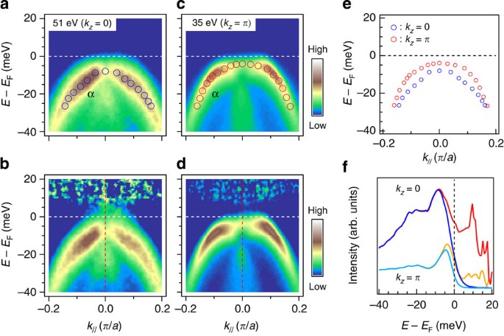Figure 3: Band dispersion of the α band atkz=0 andπin LiFe0.97Co0.03As. (a,c) show the ARPES intensity plots of LiFe0.97Co0.03As at 51 eV (kz=0) and 35 eV (kz=π), respectively. The data are recorded at 20 K with linearly polarized light to enhance the α band11,17. Blue and red circles on top of the intensity are extracted from EMDCs. (b,d) are the same data but divided by the FD function convoluted with the system resolution. (e) The extracted band dispersions froma,care plotted together and prove that the band top of the α band has tiny dispersion alongkz. (f) The EDCs at the Brillouin zone centre as marked by the red dashed line inb,d. Red and yellow curves are the same data of blue and cyan curves but divided by the FD function convoluted with the system resolution. Figure 3a,c shows the ARPES intensity plots of 3% Co at 51 eV ( k z =0) and 35 eV ( k z = π ), respectively. The data are recorded at 20 K with linearly polarized light to enhance the intensity of the α band [11] , [17] . The intensity plots and EDCs show that the band top of the α band has tiny dispersion along k z and prove that at least for 3% Co, the α band is completely sinking below E F all over the momentum space. The disappearance of the α FS reduces the density-of-states near E F and hence significantly suppresses the interband scattering between the α band and the electron FSs at the M point ( π ,0), as seen from Fig. 2m–o . Figure 3: Band dispersion of the α band at k z =0 and π in LiFe 0.97 Co 0.03 As. ( a , c ) show the ARPES intensity plots of LiFe 0.97 Co 0.03 As at 51 eV ( k z =0) and 35 eV ( k z = π ), respectively. The data are recorded at 20 K with linearly polarized light to enhance the α band [11] , [17] . Blue and red circles on top of the intensity are extracted from EMDCs. ( b , d ) are the same data but divided by the FD function convoluted with the system resolution. ( e ) The extracted band dispersions from a , c are plotted together and prove that the band top of the α band has tiny dispersion along k z . ( f ) The EDCs at the Brillouin zone centre as marked by the red dashed line in b , d . Red and yellow curves are the same data of blue and cyan curves but divided by the FD function convoluted with the system resolution. Full size image In the SC state, electrons are gapped towards higher binding energies and form a well-defined Bogoliubov quasiparticle peak. Figure 2m compares the representative EDCs of pristine LiFeAs across the Γ point above and below T c . The electronic states within the SC gap are significantly altered, while the states at higher binding energies are only slightly modified by the Bogoliubov dispersion: where E k is the energy of the Bogoliubov quasiparticle, which will not show clear deviation from the NS energy ξ k when ξ k is much larger than the SC gap Δ k . Interestingly, we find that near the band top, the electronic states of the 1% Co and 3% Co samples are slightly shifted to higher binding energies as shown in Fig. 2n,o , indicating the opening of a SC gap on the α band, even though this α band is located below E F at these doping levels ( Supplementary Fig. 3 ). Extraction of the SC gap To see how the SC condensation affects the electronic states away from E F , we show the simulated EDCs without FD distribution in the NS and SC state in Fig. 4b , corresponding to the vertical line at the Γ point in the simulated NS intensity plot in Fig. 4a . The band tops are set at 8 and 20 meV below E F , respectively, in agreement with the real band positions in this material. With a 5-meV SC gap turned on, the low-energy peak (P1) is shifted by 2 meV, while the high-energy peak (P2) is almost unchanged. Moreover, due to the particle–hole mixing, a small peak above E F develops in the EDC of the SC state. Back to the experimental data, in Fig. 4c,e,g , the EDCs at the BZ centre exhibit a coherent peak developing at all three doping levels below T c . 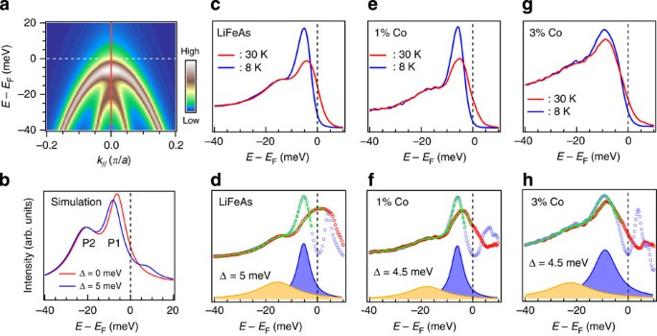Figure 4: Extracting the SC gap from EDCs. (a) ARPES intensity plot that simulates the NS band dispersion without FD distribution of 3% Co sample. (b) Simulated EDCs in the NS (red) and SC state (blue), corresponding to the vertical line in the intensity plot ina. The spectral function is assumed to have the BCS form. The small peak aboveEFin the blue EDC is due to the particle–hole mixing, which is a hallmark of SC condensation. By using the BCS spectral function to fit the EDCs in the NS and the SC state, we extract the SC gap. (c,e,g) EDCs at the BZ centre in the NS and the SC state of pristine LiFeAs, 1% Co and 3% Co samples, respectively. The EDCs are obtained by combining three EDCs near the Brillouin zone centre. To extract the SC gap, the raw data shown inc,e,gare divided by FD function convoluted with the system resolution and shown ind,f,h, respectively. Green dotted curves on light blue and red circles are the fitting results. The decomposed spectral functions in the SC state are appended below the fittings. The broadening of the decomposed peaks at higher doping levels is likely caused by an enhanced impurity scattering due to the in-plane substitution. Figure 4d,f,h shows the same data but divided by the FD function convoluted with the system resolution. To extract the SC gap, the EDCs in the NS and SC state are fitted by the BCS spectral function plus a constant background ( Supplementary Table 1 ). The extracted SC gap keeps almost constant, while the line width of the coherent peak becomes broader at higher doping levels. This indicates that the Co substitution introduces impurity potentials, which is believed to play a destructive role in sign-reversal pairing, at least in the weak coupling regime [1] . Figure 4: Extracting the SC gap from EDCs. ( a ) ARPES intensity plot that simulates the NS band dispersion without FD distribution of 3% Co sample. ( b ) Simulated EDCs in the NS (red) and SC state (blue), corresponding to the vertical line in the intensity plot in a . The spectral function is assumed to have the BCS form. The small peak above E F in the blue EDC is due to the particle–hole mixing, which is a hallmark of SC condensation. By using the BCS spectral function to fit the EDCs in the NS and the SC state, we extract the SC gap. ( c , e , g ) EDCs at the BZ centre in the NS and the SC state of pristine LiFeAs, 1% Co and 3% Co samples, respectively. The EDCs are obtained by combining three EDCs near the Brillouin zone centre. To extract the SC gap, the raw data shown in c , e , g are divided by FD function convoluted with the system resolution and shown in d , f , h , respectively. Green dotted curves on light blue and red circles are the fitting results. The decomposed spectral functions in the SC state are appended below the fittings. The broadening of the decomposed peaks at higher doping levels is likely caused by an enhanced impurity scattering due to the in-plane substitution. Full size image Following the procedure shown in Fig. 4 , we extract the low-energy band dispersion below and above T c . 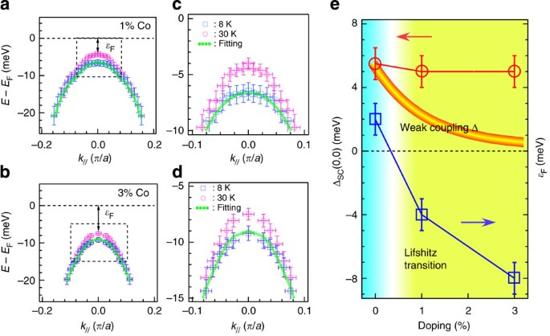Figure 5: Extraction of the SC gap from dispersions and robustness of the pairing against the disappearance of FS. (a,b) Extracted band dispersions of 1% Co and 3% Co below (light blue squares) and above (pink circles)Tc. The energy error bars are determined by the s.d. of the fitted parameters. The momentum error bars are determined by our momentum resolution times a factor of 3, since we combined three nearby EDCs to reduce the noise level. A zoom into a narrower energy range inc,dshow that the difference between the NS and the SC state is the largest at the βZ centre, and then gets smaller at high binding energies. The green dotted curves are the fitting results, which yield a similar SC gap as extracted from EDCs. (e) Comparison of the extracted SC gap from the experimental data and the expected ones from weak coupling theories. This shows that the SC gap observed on the α band is robust despite the disappearance of the α FS at the Γ point. This observation is incompatible with the weak coupling theory, in which the SC gap is expected to be sensitive to both the density-of-states nearEFand impurity scattering. Figure 5a–d show the extracted data of the 1% Co and 3% Co samples in wide and narrow energy ranges. In agreement with equation (1), the band shift is the largest near the band top and quickly vanishes at higher binding energies. By using the NS data to fit the dispersion in the SC state, we extract the SC gaps of pristine LiFeAs, 1% Co and 3% Co and plot them as a function of the Co concentration in Fig. 5e . The SC gap on the α band remains almost constant, while the associated FS topology undergoes a Lifshitz transition with the substitution of Co. Figure 5: Extraction of the SC gap from dispersions and robustness of the pairing against the disappearance of FS. ( a , b ) Extracted band dispersions of 1% Co and 3% Co below (light blue squares) and above (pink circles) T c . The energy error bars are determined by the s.d. of the fitted parameters. The momentum error bars are determined by our momentum resolution times a factor of 3, since we combined three nearby EDCs to reduce the noise level. A zoom into a narrower energy range in c , d show that the difference between the NS and the SC state is the largest at the βZ centre, and then gets smaller at high binding energies. The green dotted curves are the fitting results, which yield a similar SC gap as extracted from EDCs. ( e ) Comparison of the extracted SC gap from the experimental data and the expected ones from weak coupling theories. This shows that the SC gap observed on the α band is robust despite the disappearance of the α FS at the Γ point. This observation is incompatible with the weak coupling theory, in which the SC gap is expected to be sensitive to both the density-of-states near E F and impurity scattering. Full size image Since LiFe 1− x Co x As is a multi-orbital superconductor, the large SC gap observed on the α band, in principle, can be induced via proximity to other bands, which are crossing E F at all doping levels. In this scenario, the SC gap on the α band is expected to be smaller than the other bands and to give a negligible contribution to the SC pairing. To justify this point, we show the SC gap on the β, γ and δ bands of 3% Co in Fig. 6 . The extracted SC gap on the β, δ and γ bands are 3.3, 3.5 and 4 meV, respectively ( Supplementary Table 2 ). Since the cut on the γ band measures the largest gap on the electron FSs [15] , [16] , our results prove that the SC gap on the α band is the largest over the momentum space and thus rule out the possibility of a proximity effect causing by the pairing on other FS sheets. 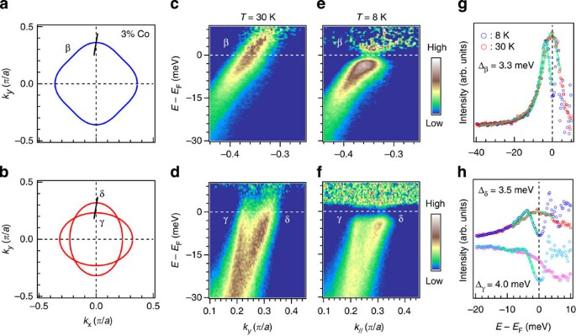Figure 6: SC gap on β and electron FSs. The measuredkFpositions are illustrated inaandb. (c–f) ARPES intensities that are divided by the FD function convoluted with the system resolution. NS and SC state EDCs that are crossed thekFpositions of the β, γ and δ bands are shown ingandh. Red/pink and blue/cyan circles represent the NS and SC state EDCs respectively. The gap values are extracted by using BCS spectral function plus a polynomial function. The fitted results are shown ingandhwith green dashed curves. Figure 6: SC gap on β and electron FSs. The measured k F positions are illustrated in a and b . ( c – f ) ARPES intensities that are divided by the FD function convoluted with the system resolution. NS and SC state EDCs that are crossed the k F positions of the β, γ and δ bands are shown in g and h . Red/pink and blue/cyan circles represent the NS and SC state EDCs respectively. The gap values are extracted by using BCS spectral function plus a polynomial function. The fitted results are shown in g and h with green dashed curves. Full size image As discussed before, the interband scattering in the particle–particle channel is dramatically reduced due to the Lifshitz transition. According to the weak coupling nesting scenarios, the SC gap on the α band is expected to exponentially decrease when the contribution of this band to the density-of-states at E F goes to zero [18] , [19] , as shown in Fig. 5e . This is clearly in contradiction with our experimental observation that the SC gap on the α band is robust and the largest over the momentum space. Recent inelastic neutron scattering and NMR studies have demonstrated that low-energy spin fluctuations are relatively weak and incommensurate for pristine LiFeAs [20] , [21] , [22] . Combined with ARPES data, the incommensurate inelastic neutron scattering peaks were attributed to the interband scattering between the β FS and the electron FSs [23] . However, ARPES and STM studies demonstrate that the largest SC gap is indeed on the α band, which is clearly incompatible with the low-energy spin fluctuations scenario [15] , [16] , [24] , [25] . Although this discrepancy can be removed by subtle modifications involving orbital fluctuations or small-q interband scattering [26] , [27] , our observation of strong SC pairing on the band without FS is beyond any reasonable mending within the weak coupling approach. Instead, it is naturally consistent with many strong coupling approaches [6] , [7] , [8] , [9] , [10] , [28] , [29] , in particular with the J 1 –J 2 model that predicts the strongest pairing at the zone centre [6] , [7] , [8] , [9] . Indeed, the ratio 2Δ α / k B T c ~7 observed in the LiFe 1− x Co x As is twice larger than the predicted BCS value, which also suggests a strong coupling pairing mechanism. Finally, it is interesting to compare the observed SC gap with ε F , here defined as the energy difference from the band top to the chemical potential [30] , as illustrated in Fig. 5a . Previous studies on the iron-chalcogenide superconductor FeTe 1− x Se x (refs 30 , 31 ) show that the SC gap is comparable with ε F and consistent with a BCS–BEC crossover scenario [29] , [30] . In LiFe 1− x Co x As, as shown in Fig. 5e , the value of ε F drops from +2 to −8 meV with 3% Co substitution, while the SC gap remains almost unchanged and is immune to the Lifshitz transition. We note that due to the multi-orbital nature of the IBSCs, the value of the Fermi energy might be much larger than we defined here, and whether the LiFe 1− x Co x As lays in the BCS–BEC crossover regime needs further experimental and theoretical investigations. Sample preparation and experimental setup Single crystals of LiFe 1− x Co x As were synthesized by the self-flux method using Li 3 As, Fe 1– x Co x As and As powders as starting materials. The Li 3 As, Fe 1− x Co x As and As powders were weighed according to the element ratio of Li(Fe 1− x Co x ) 0.3 As. The mixture was grounded and put into an alumina crucible and sealed in Nb crucibles under 1 atm of Argon gas. The Nb crucible was then sealed in an evacuated quartz tube, heated to 1,100 °C and slowly cooled down to 700 °C at a rate of 3 °C per hour. High-energy-resolution ARPES data were recorded at the Institute of Physics, Chinese Academy of Sciences, using the He Iα ( hν =21.218 eV) resonance line of a helium discharge lamp. The angular and momentum resolutions were set to 0.2° and 3 meV, respectively. ARPES polarization-dependent measurements were performed at Beamline I05 of Diamond Light Source using a Scienta R4000 with energy and momentum resolutions set to 0.2° and 10 meV, respectively. To select the α band, we employed linearly polarized light with the potential vector perpendicular to the mirror plane of the sample. All samples were cleaved in situ . The data were taken in a vacuum better than 3 × 10 −11 Torr with discharge lamp and 1 × 10 −10 Torr with synchrotron light source. Extraction of the SC gap To extract the SC gap from EDCs, we use the functions: Here we assume a BCS spectral function in the occupied states, with the Γ k parameter not changing with binding energy. a i is a fitting constant, which is proportional to Γ k and u k 2 . The fitting parameters are summarized in Supplementary Tables 1 and 2 . Equations (2)–(4), ,  are used to fit the SC gap of the α, β and γ/δ FSs, respectively. The first and second BCS spectral function in equation (2) are used to fit the α band and α′ band, respectively [11] . Since the γ and δ bands are close to each other, we use a polynomial function to remove the large background, and we assume the background has an even symmetry with respect to E F (ref. 32 ). Since the BCS spectral function can be derived from the Bogoliubov formalism, it can be applied to the strong coupling regime [31] , [33] , [34] , [35] . How to cite this article : Miao, H. et al. Observation of strong electron pairing on bands without Fermi surfaces in LiFe 1- x Co x As. Nat. Commun. 6:6056 doi: 10.1038/ncomms7056 (2015).